Correspondence: On the enzymology and significance of HSPA1 lysine methylation 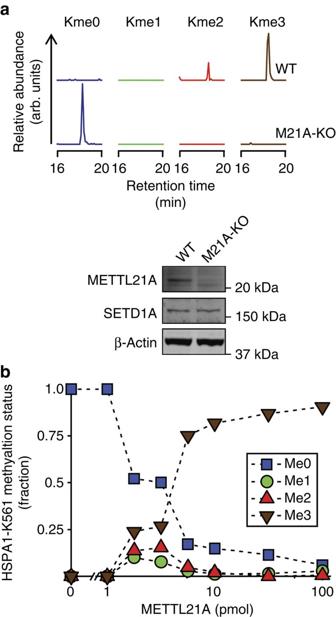Figure 1: METTL21A-mediated methylation of HSPA1-K561. (a) METTL21A knockout abrogates methylation of HSPA1-K561in vivo. Top panel, extracted ion chromatograms corresponding to mass-to-charge ratios of the various methylated forms (Kme0, Kme1, Kme2 and Kme3) of a previously studied2,4AspN-generated proteolytic peptide covering Asp555–Ala565 of HSPA1 from KBM-7 wild-type (WT) and corresponding METTL21A knock-out (M21A-KO) cells. Bottom panel, western blot analysis of METTL21A and SETD1A in cell lines analysed in the upper panel. β-Actin was used as a loading control. (b) METTL21A-mediated methylation of HSPA1-K561 is non-processive. Recombinant human HSPA1 was treated with varying amounts of METTL21A in the presence of the methyl donorS-adenosyl methionine and the relative abundance of the various methylated forms of K561 was determined by mass spectrometry. 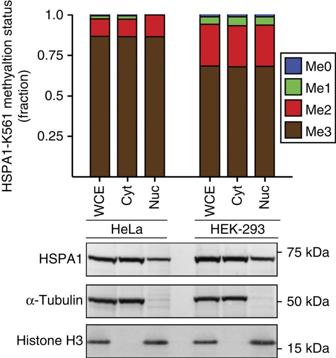Figure 2: Methylation status of HSPA1-K561 in subcellular fractions. Top panel, methylation status in whole-cell extracts (WCE) as well as in cytosolic (Cyt) and nuclear (Nuc) fractions from HeLa and HEK-293 cells was determined by mass spectrometry as inFig. 1a. Bottom panel, western blot analysis of total HSPA1, alpha-tubulin (cytosolic marker) and histone H3 (nuclear marker) in protein samples analysed in the upper panel. Cell culture and preparation of cellular protein fractions KBM-7 wild type (P00174R07) and METTL21A-gene-trapped cells (P00213G12) were purchased from Horizon Genomics (formerly Haplogen); HeLa cells were obtained from ATCC and HEK-293 cells (Flp-In T-REx 293) from Invitrogen. All cell lines were tested negative for Mycoplasma infection. KBM-7 cells were cultured in IMDM-Glutamax TM (Thermo Scientific), while HeLa and HEK-293 cells were cultured in DMDM-Glutamax TM (Thermo Scientific). All media was supplemented with 10% fetal bovine serum and 100 U ml −1 penicillin/streptomycin. Whole-cell extracts for western blot analysis of METTL21A and SETD1A protein levels were prepared by culturing cells to near confluency in a 10-cm-diameter dish, whereafter cells were harvested by scraping and collected by centrifugation at 300 g for 5 min. Cells were thereafter washed three times by dilution in 1 ml PBS and collected by centrifugation as described above. The resulting pellet was dissolved in 1% SDS, 1 mM phenylmethylsulphonyl fluoride (PMSF) (Sigma-Aldrich) and 1x protease inhibitor cocktail (Sigma-Aldrich), whereafter the protein concentration was determined with the BCA method. Subcellular fractions were prepared using a slightly modified version of the so-called rapid, efficient, and practical (REAP) method [8] . In brief, HeLa and HEK-293 cells were cultured to near confluency on 10-cm-diameter dishes. The cells were then washed with ice-cold PBS (pH 7.4), harvested by scraping, collected in 1 ml cold PBS and pelleted by centrifugation at 300 g for 5 min. The pellet was resuspended in 900 μl lysis buffer (PBS supplemented with 0.1% NP40, PMSF (Sigma-Aldrich) and protease inhibitor cocktail (Sigma-Aldrich)), whereafter a 300-μl sample representing ‘whole-cell lysate’ was removed for later analysis. The remaining sample was processed in a pop-spin centrifuge for 30 s, whereafter 300 μl of the supernatant, representing ‘cytosolic fraction’, was removed. The remaining supernatant was then removed and the pellet, representing ‘nuclear fraction’, was washed three times in lysis buffer and harvested by centrifugation as above. All fractions were then denatured in NuPAGE (Invitrogen) buffer and a normalized amount of sample was loaded on SDS-polyacrylamide gel electrophoresis (PAGE) for western blot and mass spectrometry analyses. Western blotting Twenty micrograms of protein extracts from KBM-7 cells and 30 μl ‘whole-cell extract’, and equivalent amount of cytosolic and nuclear fractions, from HeLa and HEK-293 cells were separated by SDS-PAGE and transferred to polyvinylidene difluoride membranes. Membranes were blocked overnight with 5% bovine serum albumin in Tris-buffered saline (TBS; pH 7.4), incubated with relevant primary antibodies (see below), washed three times with TBS for 10 min, incubated with appropriate horseradish peroxidase-coupled secondary antibody and finally washed six times for 10 min with TBS supplemented with 0.05% Tween. Membranes were then treated with SuperSignal™ enhanced chemiluminescent substrate (Thermo Fisher) and staining was visualized with a CCD-based imager. The following primary antibodies were used (working dilution is indicated): anti-HSPA1 (Abcam ab79852; 1:10,000), anti-METTL21A (Sigma-Aldrich HPA034712; 1:250), anti-SETD1A (Abcam ab70378; 1:1,000), anti-beta Actin (Abcam ab8227; 1:3,000), anti-alpha Tubulin (Abcam ab4074; 1:300) and anti-Histone H3 (Abcam ab1791; 1:3,000). Mass spectrometry analysis Analysis of HSPA1-Lys561 methylation events was essentially performed as previously described [2] , [4] . In brief, protein samples were separated by SDS-PAGE, whereafter the gel region encompassing HSPA1 was excised and treated with the endoprotease AspN. The resulting peptides were analysed by reverse-phase liquid chromatography coupled to a LTQ Orbitrap XL mass spectrometer (Thermo Scientific) via nanoelectrospray, using collision-induced fragmentation. Ion chromatograms corresponding to the different methylated forms of HSPA1-Lys561 were generated by gating for relevant mass-to-charge ratios of the AspN-proteolytic peptide Asp555-Ala565, z =2, of HSPA1 using Xcalibur Qual Browser (v2.0.7). The selective ion settings used were m / z =573.8037 (me0), 580.8115 (me1), 587.8193 (me2) and 594.8272 (me3)+/−10 p.p.m. The relative abundance of the different methylated species of HSPA1-Lys561 was approximated as the ratio between the area under the relevant chromatographic peak (for example, MeO, Me1, Me2 or Me3) and the sum of the area under all peaks (MeO, Me1, Me2 and Me3). The area under the peaks was determined by integration using Xcalibur Qual Browser (v2.0.7). Expression and purification of recombinant proteins The previously described [2] plasmids pET28a-METTL21A and pGEX-6p-HSPA1 were transfected into the Escherichia coli BL21-CodonPlus(DE3)-RIPL expression strain (Agilent). 6xHis tagged METTL21A and GST-tagged HSPA1 were thereafter purified using Ni-NTA agarose (Qiagen) and Glutathione Sepharose 4B (GE Healthcare), respectively, according to the manufacturer’s instructions. After affinity purification the buffer was changed to 20 mM Tris (pH 6.8), 100 mM Nacl and 1 mM DTT by sequential dilution and concentration using Vivaspin 20 ultracentrifugation columns with a molecular weight cutoff of 10 kDa (for METTL21A) or 50 kDa (for HSPA1) (Sartorius AG). Proteins were then aliquoted and stored at −80 °C and the concentration was determined using the BCA method. How to cite this article: Jakobsson, M. E. et al. Correspondence: On the enzymology and significance of HSPA1 lysine methylation. Nat. Commun. 7:11464 doi: 10.1038/ncomms11464 (2016).